Fano resonance and dipolar relaxation in lead-free relaxors Fano resonance is a phenomenon in which a discrete state interferes with a continuum of states and has been observed in many areas of science. Here, we report on the prediction of a Fano resonance in ferroelectric relaxors, whose properties are poorly understood: an ab initio molecular dynamic scheme reveals such resonance between the bare optical phonon mode of the Zr sublattice (the discrete state) and the bare optical phonon mode of the Ti sublattice (the continuum of states) in disordered lead-free Ba(Zr,Ti)O 3 . The microscopic origins of the discrete state and continuum of states are discussed in the context of relaxor properties. Furthermore, our simulations suggest that the T * characteristic temperature of relaxor is related to a hardening of the vibrational frequencies associated with fluctuation of the Ti sublattice. Finally, a terahertz relaxation mode reflecting reorientations of Ti dipoles and showing a thermally activated behaviour is predicted, in agreement with previous experiments. Canonical relaxor ferroelectrics are macroscopically centrosymmetric solid solutions or disordered compounds that are characterized by an unusually broad and frequency-dependent dielectric response versus temperature function [1] , [2] , [3] , [4] , [5] , [6] , [7] , [8] , [9] , [10] , [11] , [12] , [13] , [14] , [15] , [16] , [17] , [18] , [19] , [20] , [21] , [22] , [23] , [24] , [25] , [26] , [27] , [28] , [29] , [30] , [31] , [32] , which is often attributed to the hypothetical existence of polar nanoregions (PNRs) inside a paraelectric matrix. Relaxor ferroelectrics also typically exhibit three characteristic temperatures, known as the Burns temperature T B , freezing temperature T f and the so-called T * (refs 2 , 3 , 4 , 23 , 24 ). While it is traditionally believed that T B is associated with the formation of dynamical PNRs and that T f corresponds to the temperature at which these PNRs become static, the precise microscopic origin of the third and intermediate critical temperature (that is T *) remains unclear and is intensively debated [24] , [33] , [34] , [35] . Owing to their fundamental interest and also technological promise, relaxors have been studied by various techniques since their discoveries. For instance, they have been investigated by Raman, neutron elastic diffuse scattering, extended X-ray absorption fine structure, high-resolution tunnelling electron microscopy, piezoresponse force microscopy, phenomenology and numerical simulations [7] , [13] , [19] , [20] , [26] , [27] , [36] , [37] , [38] , [39] , [40] , [41] . On the other hand, there is an important aspect of their properties that has been much less documented because of experimental and computational challenges to overcome, that is, their terahertz (THz) dynamics [25] , [27] , [42] , [43] . As a result, several issues remain poorly understood or even unknown. For instance, can different types of alloying atoms present in a relaxor (for example, Zr and Ti in Ba(Zr,Ti)O 3 (BZT)) be associated with phonons having different dynamics? If it is indeed the case, can these different dynamics couple to each other and what is the underlying mechanism responsible for such hypothetical coupling? One may also wonder whether both alloyed sublattices, or only the one associated with the formation of PNRs (for example, Ti in BZT), exhibit relaxational modes inherent to the reorientation of dipoles? Another important challenge is to establish whether there is any inherent connection between characteristics of these phonon or relaxational modes and T *, in order to determine the driving mechanism responsible for this temperature. Obviously, answering all these questions would lead to a significant advance in our current understanding of relaxor ferroelectrics. In this study, all the aforementioned questions are addressed by investigating, analysing and comparing with experiments the complex dielectric response of disordered BZT crystal numerically obtained in the THz regime, via a combination of a first-principles-based effective Hamiltonian and a molecular dynamics (MD) technique. BZT is chosen because it is a lead-free relaxor that has already attracted a lot of attention [19] , [27] , [38] , [44] , [45] , [46] , [47] , [48] . In relaxors, most experimental works were performed in the kilohertz regime, which is (unfortunately) not accessible by our MD techniques. However, the dielectric relaxation in relaxors is typically observed in a much wider frequency interval, which is practically limited by the phonon frequencies from the high-frequency side. Because of extremely large dielectric permittivity of relaxors, the measurements in the gigahertz (GHz)–THz range are challenging, and very few experimental data are currently available. Therefore, the information that can be obtained from MD simulations is especially important. One particular feature of BZT is that it is also experimentally known [28] to demonstrate a separate relaxation mechanism at the frequencies that are in the order of a few cm −1 , which are accessible by the present simulations. BZT has also been selected because recent simulations did reveal the importance of PNRs (that are Ti rich), and the existence of all three known characteristic temperatures of relaxors (namely, T B ≃ 450 K, T * ≃ 240 K and T f ≃ 130 K) in this system [26] , [30] , [31] . In this article, we reveal the occurrence of a Fano resonance [49] between phonon modes associated with the different types of alloyed atoms. We note that Fano resonance is a general phenomenon that is rather well known in, for example, nonlinear optics and photonics, but less documented in materials science. The Fano resonance is characterized by a specific interaction between a discrete state and a continuum of states [49] , [50] , [51] , [52] , [53] . Moreover, T * is found to be the temperature below which the vibrational frequencies associated with the fluctuation of the Ti sublattice significantly harden. This manuscript also reports the existence of a thermally activated relaxational mode (as consistent with experiments [28] ) arising from the reorientation of Ti dipoles. Dielectric response The studied material with the composition of Ba(Zr 0.5 Ti 0.5 )O 3 is made of 50% of Zr and Ti ions that are randomly distributed inside a 12 × 12 × 12 supercell (8,640 atoms). The latter is periodic along the x , y and z axes, which lie along the pseudocubic [100], [010] and [001] directions, respectively. We perform effective Hamiltonian-based MD simulations [54] , [55] , [56] , [57] to obtain complex dielectric responses of disordered BZT for temperatures ranging from 10 to 1,000 K (see the Methods section). At the end of the MD simulations, the complex electric susceptibility, χ αβ ( ν ), can be obtained using the following equation [56] , [57] , [58] , [59] : where ν is the frequency while α and β define Cartesian components, V is the volume of the chosen supercell and ε 0 is the vacuum permittivity. d ( t ) is the electric dipole moment of the system at time t , and ‹...› represents thermal averages. The total electric dipole moment, d , of the system in equation (1) obviously consists of two parts d = d Zr + d Ti where d Zr (respectively, d Ti ) is the dipole moment originating from the electric dipoles centred on Zr (respectively, Ti) sites. As a result, the total dielectric response of equation (1) can be decomposed additively into three different contributions: Here, and represent the ‘sole’ contributions of the Zr-centred sites and Ti-centred sites, respectively, to the total dielectric response. On the other hand, quantifies the role of the correlations between the Zr and Ti-centred sites in that total response. Owing to the complexity of the system under investigation, we found it is more convenient and instructive to separately compute (and fit) , and rather than the total dielectric response. The latter can then be deduced by combining the fittings of , and , as shown in Fig. 1 for the imaginary part of these responses. Note that, in the following, we will focus on the isotropic component (that is, the average of the xx , yy and zz components) of each of these different dielectric responses, but will not use any notation having subscript for brevity. 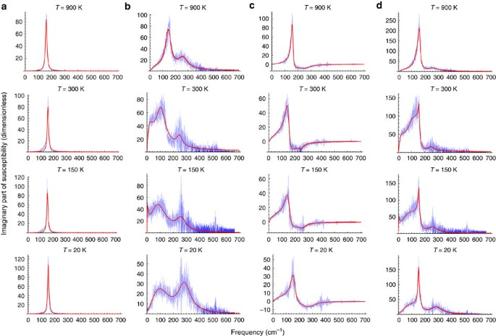Figure 1: Imaginary part of the dielectric responses of BZT as a function of frequency. (a) The dielectric response from Zr cells,χZr,Zr. (b) The dielectric response from Ti cells,χTi,Ti. (c) The dielectric response from the cross-correlation between Ti and Zr cells,χTi,Zr. (d) The total dielectric response. The solid lines in these panels represent the fitting of the MD data using analytical expressions given in equations (6) and (7), andQ(ν). The actual MD data are also shown (in blue colour) in order to confirm the adequacy of the fittings. Figure 1: Imaginary part of the dielectric responses of BZT as a function of frequency. ( a ) The dielectric response from Zr cells, χ Zr,Zr . ( b ) The dielectric response from Ti cells, χ Ti,Ti . ( c ) The dielectric response from the cross-correlation between Ti and Zr cells, χ Ti,Zr . ( d ) The total dielectric response. The solid lines in these panels represent the fitting of the MD data using analytical expressions given in equations (6) and (7), and Q ( ν ). The actual MD data are also shown (in blue colour) in order to confirm the adequacy of the fittings. Full size image Fano resonance Let us first concentrate on the MD data for the imaginary part of these different dielectric responses at T =900 K (see first row of Fig. 1 ). The imaginary part of χ Zr,Zr consists of a single narrow peak centred at ~155 cm −1 . On the other hand, both the imaginary parts of χ Ti,Ti and χ Ti,Zr exhibit anomalous features. As a matter of fact, Im( χ Ti,Ti ) appears to have two (rather than one) significant broad peaks centred at ~130 and 250 cm −1 , respectively. Similarly striking, the imaginary part of χ Ti,Zr possesses a narrow peak of ~160 cm −1 (like χ Zr,Zr ) that is followed by negative values for frequencies ranging from 200 to 300 cm −1 , which also results in the asymmetry of the lineshape ( Fig. 1c ). Interestingly, since refs. 26 , 44 indicated that PNRs (inside which Ti dipoles are parallel to each other) begin to form in BZT at the Burns temperature T B ≃ 450 K, there are no PNRs at 900 K. As a result, the anisotropy introduced by PNRs cannot be the cause of the two peaks seen in Im( χ Ti,Ti ) at 900 K. A mechanism that does not involve PNRs must therefore be responsible for the unusual features of χ Ti,Ti and χ Ti,Zr . Here, we take advantage of the insight brought by our simulations to reveal that a Fano resonance naturally explains such unusual features. For that, let us consider two linearly coupled damped harmonic oscillators (DHOs)—one of them (with bare frequency ν Ti,0 and bare damping constant Γ Ti,0 ) representing the intrinsic, bare dynamical response of the Ti sublattice, and the other (with bare frequency ν Zr,0 and bare damping constant Γ Zr,0 ) representing the intrinsic, bare dynamical response of the Zr sublattice. The dynamics of the coupled system can be described by a 2 × 2 Green’s function G ( ν )=( D − iν Γ − ν 2 I ) −1 (refs 57 , 60 ) where I is the 2 × 2 unit matrix, while the real dynamical matrix D and the real damping parameter matrix Γ read These matrices contain off-diagonal terms Δ Ti,Zr and Γ Ti,Zr describing the bilinear coupling between the Ti and Zr sublattices. Contributions to the complex dielectric susceptibility spectrum χ ( ν ) of this coupled system can be expressed via (bare) plasma frequencies Ω Ti,0 and Ω Zr,0 (for example, ref. 61 ), associated with the total dipole moment of the Ti and Zr subsystems, respectively, as , , and . Within this coupled DHOs model, the bare dielectric susceptibilities of the Zr and Ti oscillators ( ) are given by and , which can also be expressed in terms of the (perturbed) partial susceptibilities as and . Application of this model to the simulated dielectric response at 900 K is shown in Fig. 2 as an example. In this case, the parameters entering χ Zr,Zr and χ Ti,Ti , which best fit the MD results of χ Zr,Zr and χ Ti,Ti simultaneously (shown in Fig. 2a,b ), respectively, are such as: (i) the bare Zr oscillator is described by Ω Zr,0 =450 cm −1 , ν Zr,0 =170 cm −1 and Γ Zr,0 =19 cm −1 ; (ii) the bare Ti oscillator is described by Ω Ti,0 =1,250 cm −1 , ν Ti,0 =193 cm −1 and Γ Ti,0 =205 cm −1 ; and (iii) the coupling constants are Δ Ti,Zr =−8,435 cm −1 and Γ Ti,Zr =−41 cm −1 . The resulting bare χ 0 Zr,Zr and χ 0 Ti,Ti , associated with these parameters, are shown in Fig. 2d . Note that these Ω Ti,0 and Ω Zr,0 plasma frequencies correspond well to anticipated dynamical charge associated with the Ti and Zr sublattices of the effective Hamiltonian model. Furthermore, it is important to realize that the bare Ti oscillator is clearly much more damped than the Zr one. One therefore recovers a broad spectrum for the bare Ti subsystem overlapping with the resonant bare response of the Zr subsystem. From these comparisons, it is clear that the two asymmetric peaks in χ Ti,Ti are indeed caused by an interaction between the Ti and Zr subsystems. Note that the difference between Γ Ti,0 and Γ Zr,0 is compatible with the Fano resonance mechanism, that is, the broad bare Ti response provides the background component while the sharp bare Zr response provides the discrete state, the two ingredients for the Fano resonance. To understand such difference at a microscopic level, let us recall that ref. 26 revealed that Zr ions are close to their ideal cubic positions, leading to a very narrow peak in their bare dielectric response. On the other hand, the Ti ions move away from the ideal cubic positions and have an underlying anharmonic potential, with the amplitude of these motions depending on the chemical environment. As a result, the bare dielectric response of the Ti sublattice has a broad peak. Note also that the difference in the amplitude of the motions between the Zr and Ti ions was precisely found to be the origin of the formation of PNRs in disordered BZT [26] . In other words, the Fano resonance and the characteristic quantities of relaxors are found to have the same microscopic origin in our investigated disordered solid solution. Note, however, that some other properties of relaxors, such as the dependence of their susceptibility versus temperature function on frequency, are likely caused by the existence of relaxational modes (associated, for example, with dipolar dynamics of PNRs), and are thus not directly related to the Fano resonance since the latter involves phonon modes. 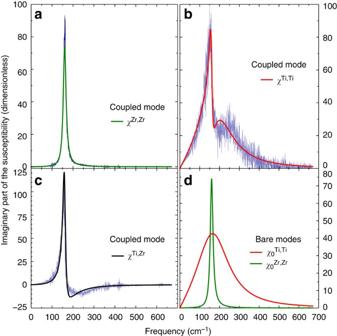Figure 2: Imaginary part of different dielectric responses of BZT as a function of frequency atT=900 K. (a–c) The dielectric responses from Zr cells,χZr,Zr, from Ti cells,χTi,Ti, and from the cross-correlation between Ti and Zr cells,χTi,Zr, which include the coupling between the bare responses of Ti and Zr sublattices. (d) The bare dielectric response from Zr cells,χ0Zr,Zrand bare dielectric response from Ti cells,. The actual MD data are also shown (in blue colour) in order to confirm that Fano interference leads to the main striking features adopted byχTi,TiandχTi,Zr. The parameters entering this interference are found by simultaneously fitting the MD data ofχTi,TiandχZr,Zrusingand. Figure 2: Imaginary part of different dielectric responses of BZT as a function of frequency at T =900 K. ( a – c ) The dielectric responses from Zr cells, χ Zr,Zr , from Ti cells, χ Ti,Ti , and from the cross-correlation between Ti and Zr cells, χ Ti,Zr , which include the coupling between the bare responses of Ti and Zr sublattices. ( d ) The bare dielectric response from Zr cells, χ 0 Zr,Zr and bare dielectric response from Ti cells, . The actual MD data are also shown (in blue colour) in order to confirm that Fano interference leads to the main striking features adopted by χ Ti,Ti and χ Ti,Zr . The parameters entering this interference are found by simultaneously fitting the MD data of χ Ti,Ti and χ Zr,Zr using and . Full size image Moreover, and as further evidenced in Fig. 2c (that displays the cross-function χ Ti,Zr , resulting from the aforementioned coupled DHO model and parameters, along with the actual MD data), the motions of the Ti and Zr ions become coupled to each other as a result of this Fano coupling. One can clearly see that the asymmetry and negative values of χ Ti,Zr , are all well reproduced by the fitting, which further emphasizes the relevance of the Fano resonance in BZT relaxors. Note that a Fano resonance has also been recently suggested to have a role in the (K 1− x Li x )TaO 3 relaxor ferroelectric [53] . However, this resonance is different from ours and rather complex, since it is proposed to involve normal modes (corresponding to different discrete oscillating configurations) of the whole nanocomposite (that is, made of the polar nanodomains and the host matrix) that are coherently coupled to each other via a piezoelectrically assisted relaxation continuum. Similarly, the Fano resonances observed in the non-relaxor LiNbO 3 material [51] are certainly of different nature. In contrast, our proposed Fano resonance simply consists of two coupled optical phonon modes. To further demonstrate that the proposed Fano resonance occurs in BZT relaxors, we performed additional MD simulations in which the resonance of χ Zr,Zr is artificially tuned to 450 cm −1 , which is far away from the (bare) resonance of χ 0 Ti,Ti . In such a case, we numerically found that, for example, χ Ti,Ti has now only one (broad) peak rather than two, which confirms once again the adequacy of the Fano interference in our investigated system. The aforementioned simple model, based on a Fano interference between the bare DHO modes of the Zr and Ti sublattices, therefore allows us to understand and reproduce all the striking features of the perturbed dielectric spectra (that is, the single sharp peak of χ Zr,Zr , the double broad peaks of χ Ti,Ti , and the asymmetry and negative values of χ Ti,Zr ). However, as shown in Fig. 2 , this model does not ‘perfectly’ fit the MD data over the entire range of investigated frequencies. For instance, the second (highest-in-frequency) peak of χ Ti,Ti could be better described between ≃ 200 and 300 cm −1 . We numerically found that such slight imperfection is related to the atomic disorder existing inside our investigated system. This fact is evidenced by further simulations ( Supplementary Note 1 ) we conducted at 900 K on a perfectly rocksalt-ordered realization of BZT in which the Zr and Ti ions alternate along any Cartesian direction (note that this rocksalt ordering is possible to create when the overall Zr and Ti compositions are both equal to 0.5, as we choose here). In that case, coupling of the single DHOs for the bare responses of the Zr and Ti sublattices leads to an excellent fitting of the MD data ( Supplementary Fig. 1 ). Let us now investigate the χ Zr,Zr , χ Ti,Ti and χ Ti,Zr of the disordered BZT material for all temperatures, not only for high temperatures (~900 K), for which the aforementioned Fano model is enough to reproduce and understand the MD data. We (empirically) found that these dielectric responses can, in fact, be reasonably well fitted for any temperature by different analytical expressions, which we now report and discuss. The sole contribution of the Zr-centred sites, χ Zr,Zr , can be well fitted by a single DHO of the form: where ν Zr–Zr is the resonant frequency, Ω Zr is the plasma frequency and γ Zr–Zr is the damping constant of this mode. Note that Ω Zr is numerically found to be approximately a constant independent of temperature, as consistent with the anticipated dynamical charge associated with the Zr sublattice of the effective Hamiltonian model. The result of this fitting of the imaginary part of χ Zr,Zr is shown in Fig. 1a for four representative temperatures, which are T =900, 300, 150 and 20 K, showing a narrow peak for any of these temperatures. Regarding χ Ti,Ti , we decided to use two DHOs and also a Debye mode for any temperature. The necessity of two DHOs for χ Ti,Ti fitting is a consequence of the aforementioned Fano coupling between the bare DHO modes of Zr and Ti sublattices. The introduction of the Debye mode was deemed necessary in order to describe the low-frequency peak that can be clearly seen in Fig. 1b for the 300 and 150 K data. It does not originate from, nor is involved in, the presently discovered Fano coupling, unlike the Fano mechanism proposed in (K 1− x Li x )TaO 3 (ref. 53 ). As we will show later, it is rather related to the flipping of Ti dipoles, which is typical of the so-called central mode [56] , [57] . We thus have: where τ Ti–Ti and are the relaxation time and static susceptibility of the Debye mode, respectively. ν Ti–Ti, i , Ω Ti–Ti, i and γ Ti–Ti, i represent the resonant frequency, plasma frequency and damping constant of the Ti-DHO mode i (with i =1 or 2), respectively. The notation i =1 (respectively, i =2) corresponds to the DHO mode having the smallest (respectively, largest) resonant frequency. 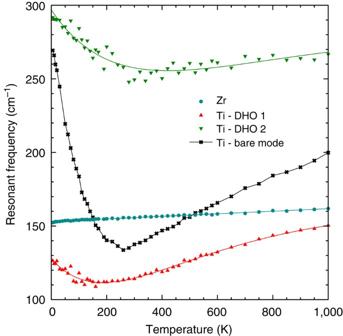Figure 3: Resonant frequencies of the DHO modes associated with the Zr and of Ti sublattices as a function of temperature. These modes correspond to the Zr-DHO mode, the Ti-DHO mode 1, the Ti-DHO mode 2 and the bare Ti-mode. Figure 3 reports the temperature evolution of the resonant frequencies of all the DHO modes associated with the Zr and Ti dielectric responses, as well as the bare resonant frequency ν Ti,0 associated with (note that the bare resonant frequency ν Zr,0 associated with is very similar to ν Zr–Zr , and is thus not shown for clarity). The resonant frequency ν Zr–Zr very slightly varies between 160 and 152 cm −1 when the temperature decreases. ν Ti–Ti,1 ranges from 110 to 150 cm −1 for the investigated temperature window. ν Ti–Ti,2 only slightly decreases when decreasing the temperature down to ~240 K, and then significantly increases from 250 to 300 cm −1 as the temperature is further decreased. Interestingly, the existence of the three predicted DHO modes for the perturbed responses, as well as the value and temperature behaviours of their resonant frequencies shown in Fig. 3 , is rather consistent with the experimental work on Ba(Zr 0.4 Ti 0.6 )O 3 (ref. 27 ), revealing the existence of two modes at ~100 and 140–150 cm −1 that are nearly independent of temperature and a third phonon mode at 200 cm −1 whose resonant frequency increases when the temperature decreases below 250 K. According to our simulations, such modes correspond to the Ti-DHO mode 1, the DHO mode of Zr ions and the Ti-DHO mode 2, respectively (note, however, that there is a subtle difference between the measurements and simulations, in the sense that the experiments indicate that the lowest transverse optical phonon mode of Zr ions and Ti ions should be of the Last and Slater type, respectively [27] , while the simulations lead to an intermediate situation between the Last and Slater types for the three aforementioned DHOs by construction of the effective Hamiltonian, see the Methods section). Figure 3 further reveals that the noticeable non-monotonic behaviour of ν Ti–Ti,2 at ~240 K originates from a striking enhancement of the bare resonant frequency ν Ti,0 below such temperature. Remarkably, 240 K is the previously predicted value of the so-called T * characteristic temperature [24] of BZT [26] . Moreover, the average magnitude of the Ti dipoles was found to significantly increase when decreasing the temperature below T * in ref. 26 , which bears resemblance to the enhancements of ν Ti–Ti,2 from 250 to 300 cm −1 and of ν Ti,0 from 130 to 270 cm −1 depicted in Fig. 3 . This controversial characteristic temperature T * therefore appears to be associated with a hardening of a very specific sublattice, namely the Ti sublattice. It will be interesting in the future to determine whether this is the case for other relaxors, since recent works seem to indicate that T * may have a different origin between lead-free and lead-based relaxors [33] , [34] , [35] . Figure 3: Resonant frequencies of the DHO modes associated with the Zr and of Ti sublattices as a function of temperature. These modes correspond to the Zr-DHO mode, the Ti-DHO mode 1, the Ti-DHO mode 2 and the bare Ti-mode. Full size image Dipolar relaxation As indicated in equation (7), χ Ti,Ti also possesses a relaxation mode in addition to these two DHO modes. Microscopically, the existence of DHOs and Debye mode is because of the pronounced multipotential well structure for the dipoles on Ti sites: DHO modes are typically related to oscillations of Ti ions inside potential wells, whereas the Debye mode is associated with the hopping of Ti ions among the off-centred sites, which is also known as the central mode [56] , [57] . This relaxation mode is denoted as R Ti–Ti in the following. As shown in Fig. 4a , the Debye frequency of R Ti–Ti (that is, 1/ τ Ti–Ti ) decreases from ~60 cm −1 to nearly zero when the system is cooled down from 1,000 K to the lowest investigated temperatures (note that these low frequencies imply that the relaxational Ti mode does not overlap with the Zr bare DHO mode, therefore preventing a Fano coupling between these two modes). 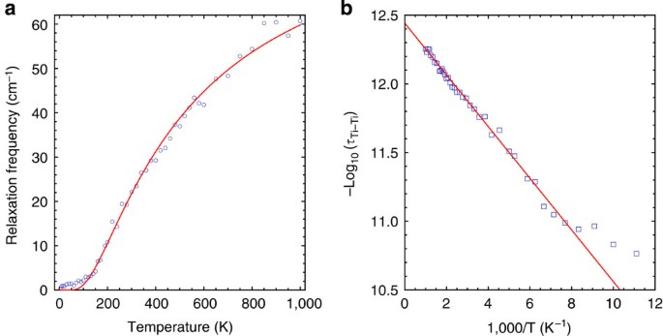Figure 4: Temperature dependence of the Debye frequency associated with theRTi–Tirelaxational mode of Ti ions. (a) The dependence in linear scales is shown ina, while inbsuch frequency is shown in logarithmic scale withτTi–Tibeing in unit of second, and as a function of the ratio of 1,000 and the temperature (expressed in Kelvin). The solid line in both panels corresponds to the fitting by an Arrhenius law, 1/τTi–Ti=ν0exp(−U/kBT). Figure 4b clearly shows that this frequency follows an Arrhenius law, 1/ τ Ti–Ti = ν 0 exp(− U / k B T ), with ν 0 ≃ 2.8 THz and the activation energy, U ≃ 0.038 eV, when the temperature is above ~130 K. Interestingly, a thermally activated process with an activation energy of the same order of magnitude was indeed observed experimentally in the THz spectra of Ba(Zr 0.4 Ti 0.6 )O 3 (ref. 28 ), which further attests the validity of our simulations (more precisely, the observed THz relaxation mode has been quantitatively evaluated in an unpublished work by the authors of ref. 28 for temperatures ranging from 300 to 700 K, and can be described by an Arrhenius law with an estimated activation energy of 0.07 eV and a limiting frequency of 1 THz). It is also worthwhile to note that Fig. 4 seems to indicate that the relaxation time of R Ti–Ti deviates from the Arrhenius law below 130 K. This temperature was found in ref. 26 to be the characteristic temperature, T f , that signals the formation of (larger) static PNRs, all having a polarization being aligned along one of the eight possible ‹111› pseudocubic directions (note that T f was practically determined to be the temperature at which the static dielectric response peaks, and was termed as the freezing temperature in ref. 26 . This denomination of freezing temperature has to be taken with a grain of salt, since the traditional definition of a freezing temperature for relaxors is technically different: it is rather the non-zero temperature appearing in the Vogel–Fulcher law for which the relaxation time tends to be infinite [4] ). However, one has also to realize that the relaxation frequency of R Ti–Ti below 130 K begins to become close to the limiting minimal values that are technically accessible by our MD simulations (estimated to be ~0.3 cm −1 ). An experimental validation of our prediction of a change in Arrhenius behaviour of R Ti–Ti around T f is therefore needed before asserting that this is not an artefact of the MD simulations. Let us also indicate that, at frequencies below GHz range (which are technically inaccessible in our simulations), another thermally activated relaxation following the Arrhenius behaviour was experimentally revealed for T < T B [27] , [28] . This relaxation was found to be independent of the Ti concentration in the BZT solid solutions and to possess a somewhat higher activation energy of U ≃ 0.167 eV (refs 27 , 28 ). In contrast to R Ti–Ti that is associated with reorientations of individual dipoles in Ti cells, we believe that the lowest in-frequency relaxation mode may originate from the collective dynamics inside PNRs or even thermally activated reorientations of the whole PNRs [3] , [4] . Figure 4: Temperature dependence of the Debye frequency associated with the R Ti–Ti relaxational mode of Ti ions. ( a ) The dependence in linear scales is shown in a , while in b such frequency is shown in logarithmic scale with τ Ti–Ti being in unit of second, and as a function of the ratio of 1,000 and the temperature (expressed in Kelvin). The solid line in both panels corresponds to the fitting by an Arrhenius law, 1/ τ Ti–Ti = ν 0 exp(− U / k B T ). Full size image We now briefly discuss the dielectric response, χ Ti,Zr , obtained from the cross-correlation of Zr and Ti sites ( Fig. 1c ). As discussed above, the unusual striking features of Im( χ Ti,Zr ), including the negative values in some frequency range and its asymmetric lineshape, can be qualitatively well understood by considering a Fano resonance between the bare response of the Zr sublattice and the bare response inherent to the Ti sublattice. Practically, the following phenomenological expression (which is adapted from the original equation proposed by Fano himself [49] ) was found necessary to adequately fit the MD data, in general, and quantitatively reproduce such subtle and fine features, in particular, , where ν 0 is the resonance frequency, γ res describes the linewidth and q res is the Fano parameter determining the asymmetry of the lineshape of the resonance, which is traditionally understood as a ratio between the rates of two transition pathways: one for the direct transition to the discrete state and the other for the two-step transition to the discrete state via the continuum [62] . Note that the −1 appearing in the bracket is inserted here in order to exclude the background continuum response. Finally, Q 0 ( ν ) typically represents the unperturbed, but nonuniform, continuum background absorption [63] . Q 0 ( ν ) therefore originates from the Ti dipoles and, thus, can be represented by a Debye and a DHO mode, that is, Note that equation (8) represents the absorption spectra of the bare Ti contribution, that is, the broadband Ti resonance that is not affected by the interaction with the Zr sublattice. As a result, the parameters of equation (8) differ from those of equation (7), since the latter describes the perturbed response. The difference between the bare and perturbed responses of the Ti sublattice is further emphasized when realizing that two DHOs are used in equation (7) versus a single one in equation (8). We numerically found that the fitting of χ Ti,Zr by Q ( ν ) is rather good for all the available temperatures (as shown in Fig. 1c ). It is also interesting to point out that modifications of the Fano resonance, which bear resemblance to the expressions of Q ( ν ) and Q 0 ( ν ) here, were also proposed in ref. 52 . In summary, we obtained and analysed the THz dielectric response of Ba(Zr 0.5 Ti 0.5 )O 3 relaxors by decomposing it into its constitutional parts that are defined by equations (2, 3, 4). This decomposition and the analysis via the coupled DHO model using Green’s function allow us to reveal the existence, at any temperature, of a Fano resonance between the bare discrete, sharp DHO mode associated with the Zr sublattice and the bare broad DHO mode inherent to the Ti sublattice. Such difference in broadness between the bare DHO modes of the Zr versus the Ti sublattices originates from the fact that Zr ions energetically prefer to stay close to their ideal positions while Ti ions want to move off-centre with the amplitude of their motions being influenced by their environment. This difference in off-centering is precisely the reason found in ref. 26 to explain why the disordered BZT possesses PNRs and is a relaxor. It is expected that the presently discovered Fano resonance may also occur in other solid solutions whose relaxor properties arise from such difference in off-centering between their alloyed elements. Note, however, that lead-based relaxors (for example, the Pb(Mg 1/3 Nb 2/3 )O 3 -based systems), which are likely more complicated than lead-free relaxors, may need to invoke rather complex phenomena to reproduce their properties [64] . Our simulations also predict a thermally activated THz relaxation mode, which is in agreement with the previous experiment [28] . Finally, the phonon mode of the Ti sublattice hardens upon cooling through the T * temperature that is known to exist in relaxors. We therefore hope that the present work is beneficial to better understand relaxors. Effective Hamiltonian The effective Hamiltonian for BZT used here has been developed in ref. 26 and has been shown to reproduce many finite-temperature relaxor properties of this material [26] , [30] , [31] . Its internal energy is: where u i is the local soft-mode in unit cell i , which is directly proportional to the local electric dipole moment in that cell. u i is centred on the B-sites (Zr or Ti) and represents the collective motion of Ba, Zr/Ti and oxygen atoms inside this cell. { σ j } characterizes the atomic arrangement, that is σ j =+1 or −1 corresponds to the presence of a Zr or Ti atom located at the lattice site j , respectively [65] . The v ’s are Ba-centred dimensionless local displacements that are related to the inhomogeneous strain inside each cell [66] . η H is the homogeneous strain tensor [66] . The internal energy of equation (9) has two parts. The first part mimics the energetics of an hypothetical, simple Ba‹ B ›O 3 crystal in which ‹ B › is a virtual atom that can be thought as a chemical average of Zr and Ti atoms [65] , [66] , [67] . This first term collects energies related to local mode self-energy, short-range and long-range interactions between local modes, as well as elastic energy and the couplings between local modes and strains [66] . The second part is explicitly related to alloy effects on physical properties. It includes the on-site effects resulting from the difference in harmonicity between the Zr and Ti ions (this difference was found to be crucial to reproduce and understand relaxor behaviour in BZT [26] , [30] ), as well as intersite effects such as random fields and strains arising from the distribution of the Zr and Ti ions inside the supercell. All the parameters entering the analytical expression of E int are determined by performing first-principle calculations [67] , [68] , [69] , [70] on relatively small supercells (typically, <20 atoms). Practically, the PNRs are obtained by using a computer programme that examines the dipole at each Ti site to determine whether it belongs to a PNR [30] , [31] . Molecular dynamics In order to obtain the dynamical properties of BZT, the E int internal energy of equation (9) is used in MD simulations (rather than in Monte–Carlo simulations as in refs 26 , 30 , 31 ), with its degrees of freedom obeying Newton’s equation [56] : where A γ is one (Cartesian or Voigt) component of the aforementioned local modes or strains and M Aγ has a dimension of a mass. During the MD simulations, the temperatures of all these structural degrees of freedom are controlled by Evans–Hoover thermostats [56] , [59] . For each MD simulation, we first run 10 5 MD steps of NPT (isothermal–isobaric ensemble) simulations to equilibrate the system at a chosen temperature and pressure. Then, the equilibration of the system within an NVE (microcanonical) ensemble is performed through 10 5 MD steps. Subsequent 4.3 × 10 6 NVE steps are performed to obtain the time-resolved physical properties of the system. How to cite this article: Wang, D. et al . Fano resonance and dipolar relaxation in lead-free relaxors. Nat. Commun. 5:5100 doi: 10.1038/ncomms6100 (2014).